In-cell NMR reveals potential precursor of toxic species from SOD1 fALS mutants Mutations in the superoxide dismutase 1 (SOD1) gene are related to familial cases of amyotrophic lateral sclerosis (fALS). Here we exploit in-cell NMR to characterize the protein folding and maturation of a series of fALS-linked SOD1 mutants in human cells and to obtain insight into their behaviour in the cellular context, at the molecular level. The effect of various mutations on SOD1 maturation are investigated by changing the availability of metal ions in the cells, and by coexpressing the copper chaperone for SOD1, hCCS. We observe for most of the mutants the occurrence of an unstructured SOD1 species, unable to bind zinc. This species may be a common precursor of potentially toxic oligomeric species, that are associated with fALS. Coexpression of hCCS in the presence of copper restores the correct maturation of the SOD1 mutants and prevents the formation of the unstructured species, confirming that hCCS also acts as a molecular chaperone. In-cell NMR represents a unique tool for characterizing physiological processes and their alteration in the ‘natural’ environment, that is, within a live cellular context, with an atomic-level approach [1] , [2] , [3] , [4] , [5] , [6] , [7] , [8] , [9] . This level of characterization is necessary to understand the molecular cause of cell malfunction in pathological states and to develop treatments and therapeutic protocols. We have recently developed an in-cell NMR approach aimed at obtaining information directly in live human cells on the folding and maturation process of proteins as they are produced [10] , [11] . This in-human-cell NMR approach was applied to monitor maturation events for human proteins such as Mia40 (ref. 11 ) and superoxide dismutase 1 (SOD1) [10] . The latter is a stable dimer binding a catalytic copper ion and a structural zinc ion per monomer, and forming an intramolecular disulfide bond. The acquisition of one zinc ion per monomer is required for the protein to interact with its specific chaperone CCS [12] , which transfers copper to SOD1 and catalyses the disulfide bond formation, forming the mature and active SOD1 dimer [13] , [14] , [15] . SOD1 is strongly implicated in the onset of amyotrophic lateral sclerosis (ALS), an adult-onset neurodegenerative disease characterized by the death of motor neurons in the brain and spinal cord. While the majority of ALS cases are sporadic with no known aetiology, the remaining cases are genetic in origin and classified as ‘familial’ (fALS). In 1993, it was discovered that about 20% fALS cases could be related to mutations in the SOD1 gene [16] . One hundred and sixty-five unique fALS-linked SOD1 mutations have been identified so far, which are scattered throughout SOD1 amino acid sequence (ALSod, the Amyotrophic Lateral Sclerosis Online Genetic Database, 2012, http://alsod.iop.kcl.ac.uk/ ). The pathogenic role of SOD1 in ALS has been linked to the formation of protein aggregates rich in SOD1, observed both in the spinal cords of patients with ALS [17] , [18] , [19] and of transgenic mice expressing human forms of the protein [20] , [21] , [22] , [23] , with accumulation primarily in the late stages of the disease. The precursors of these protein aggregates are believed to be soluble oligomeric intermediates of the SOD1 aggregation process. These oligomers are thought to be responsible for the toxic gain of function, similar to what has been proposed for other neurodegenerative diseases [24] , [25] , [26] , [27] . Generation of soluble oligomers was found to occur through oxidation of the two free cysteines of SOD1 (C6 and C111) [28] , [29] , as well as through other possible mechanisms [30] , [31] , which give rise to various aggregation products [32] , [33] , including amyloid-like structures [34] , [35] . The mature form of SOD1 is not prone to aggregation, whereas the early species of the maturation process (that is, SOD1 lacking metal ions) have been shown to have tendency to oligomerize in vitro [28] , [36] , [37] , [38] . Therefore, an impaired maturation process would lead to the accumulation of immature SOD1 species, which are prone to oligomerization. Recent studies reported a higher propensity for deficient protein maturation in vivo or in-cell culture models for some fALS mutants [39] , [40] . However, most of the studies addressing the properties of fALS SOD1 mutants and their effects on the maturation process have been performed in vitro , therefore, far from physiological conditions [41] , [42] , [43] . In this work, the maturation process of a set of fALS mutants was studied through the in-human-cell NMR approach, already successfully applied to wild-type (WT) hSOD1 (ref. 10 ). With this approach, proteins are overexpressed and isotopically labelled in cultured human cells, and information on the intracellular folding, cysteine oxidation and metallation state of the protein is obtained by observing them directly in living cells by NMR. The maturation levels of fALS mutants in different cellular conditions (for example, different levels of copper and/or zinc and coexpression of human CCS, hCCS) were compared with those of WT hSOD1. The CCS-dependent maturation of the same set of fALS mutants was also examined through in vitro NMR experiments following the same procedure applied to WT hSOD1 (ref. 15 ). These two approaches (in-cell and in vitro NMR) allowed us to monitor each step of the fALS mutants maturation process, providing atomic-level information on how each mutation affects the ability of intracellular hSOD1 to reach its mature, stable state. We identified an unstructured species for many of the fALS mutants overexpressed in human cells. This species was not observed when the same fALS mutants were coexpressed with hCCS in the presence of copper. This unstructured species may be a common precursor to potentially toxic oligomeric species, or other aggregation products, that are associated with fALS. Selected fALS-linked SOD1 mutants A number of fALS-linked SOD1 mutations distributed over the protein structure was investigated ( Fig. 1 ). 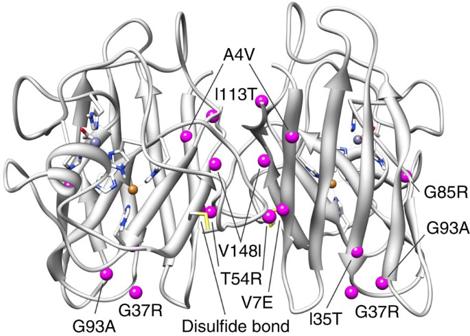Figure 1: Location of the studied fALS mutations of SOD1. The backbone positions of the studied fALS-linked mutations (magenta spheres) are displayed on the solution NMR structure of Cu(I),Zn-SOD1SS(PDB code: 1L3N), shown in white cartoon. With the exception of G85R, all the mutations reside far from the metal binding sites (shown as sticks). Copper and zinc ions are shown as orange and grey spheres, respectively. The side chains of Cys57 and Cys146 are also shown as yellow sticks. We selected the mutants A4V, V7E, G37R, T54R, G85R, G93A, I113T and V148I, featuring various properties as summarized in Table 1 . We also selected a mutation (G85R) that destabilizes the zinc-binding site [44] , and a SOD1 mutation not currently linked to fALS (I35T), but which is reported to promote SOD1 aggregation [34] . With the exception of G85R, all the selected mutations occur far from the metal binding sites. Figure 1: Location of the studied fALS mutations of SOD1. The backbone positions of the studied fALS-linked mutations (magenta spheres) are displayed on the solution NMR structure of Cu(I),Zn-SOD1 SS (PDB code: 1L3N), shown in white cartoon. With the exception of G85R, all the mutations reside far from the metal binding sites (shown as sticks). Copper and zinc ions are shown as orange and grey spheres, respectively. The side chains of Cys57 and Cys146 are also shown as yellow sticks. Full size image Table 1 Properties of the hSOD1 mutations studied in the present work. Full size table Impaired zinc binding causes accumulation of mutant apo-SOD1 The SOD1 mutants were overexpressed in HEK293T cells, transfecting them with the same amount of DNA for all the mutants. The amounts of soluble mutant proteins in the cell extracts ranged from 36±8 μM (s.d.) (G85R SOD1) to 162±8 μM (s.d.) (T54R SOD1), compared with 150 μM WT SOD1 expressed in the same conditions. For each mutant, the total amount of intracellular SOD1 was the same as that of the soluble SOD1, indicating that no significant formation of insoluble aggregates occurred to any of the mutants in these cellular conditions ( Supplementary Fig. 1 ). In absence of added metal ions, all mutants appear to lack a defined conformation, similar to what was observed for WT SOD1 expressed in the same conditions, where the in-cell NMR spectra show mainly peaks in the 8.0–8.3 p.p.m. ( 1 H) region ( Supplementary Fig. 2 ). When cells were supplemented with ZnSO 4 , even in excess, most of the fALS mutants remained predominantly unstructured ( Fig. 2 ). Specifically, for A4V, I35T, G37R, G85R, G93A and I113T SOD1 mutants, a small amount of zinc-bound protein (E,Zn-SOD1) was observed, ranging from ~5% for G85R to ~40% for G37R ( Supplementary Fig. 3 ). On the contrary, V7E, T54R and V148I SOD1 mutants stoichiometrically bound one Zn 2+ ion per monomer, and only the folded, homodimeric E,Zn-SOD1 forms were present ( Fig. 3 ), as observed for WT SOD1 (ref. 10 ). Chemical shift analysis shows that for the latter mutants only minor changes occur in the two-dimensional (2D) NMR spectra, indicating that the overall structure is maintained in the E,Zn-SOD1 form, as the mutations only cause small local perturbations on the protein conformation ( Supplementary Fig. 4 ). 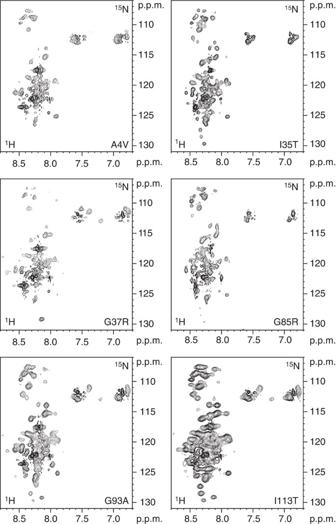Figure 2: Some fALS SOD1 mutants fail to bind zinc in the cell. 1H–15N SOFAST HMQC spectra acquired on human cell samples expressing uniformly15N-labelled SOD1 mutants in Zn(II)-supplemented medium. Most of the fALS-linked SOD1 mutants do not bind zinc when expressed, even with excess zinc in the cell culture, and an unstructured apo form accumulates in the cytoplasm. In some cases, a small amount of E,Zn-SOD1 species is also present (seeSupplementary Fig. 3). Figure 2: Some fALS SOD1 mutants fail to bind zinc in the cell. 1 H– 15 N SOFAST HMQC spectra acquired on human cell samples expressing uniformly 15 N-labelled SOD1 mutants in Zn(II)-supplemented medium. Most of the fALS-linked SOD1 mutants do not bind zinc when expressed, even with excess zinc in the cell culture, and an unstructured apo form accumulates in the cytoplasm. In some cases, a small amount of E,Zn-SOD1 species is also present (see Supplementary Fig. 3 ). 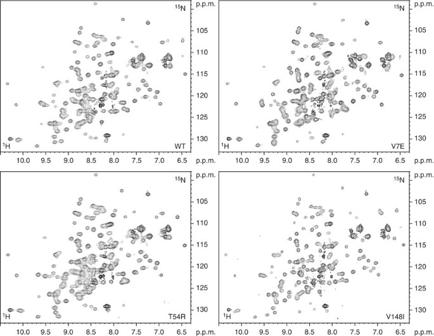Figure 3: Some fALS SOD1 mutants behave like WT SOD1. 1H–15N SOFAST HMQC spectra acquired on human cell samples expressing uniformly15N-labelled WT SOD1 and mutants in zinc-supplemented medium. A subset of the fALS-linked SOD1 mutants behave like WT SOD1, and stoichiometrically bind one zinc ion per monomer, when present in excess in the cell culture. The very small chemical shift differences between WT and mutant SOD1 indicate high structural similarity (seeSupplementary Fig. 4). Full size image Figure 3: Some fALS SOD1 mutants behave like WT SOD1. 1 H– 15 N SOFAST HMQC spectra acquired on human cell samples expressing uniformly 15 N-labelled WT SOD1 and mutants in zinc-supplemented medium. A subset of the fALS-linked SOD1 mutants behave like WT SOD1, and stoichiometrically bind one zinc ion per monomer, when present in excess in the cell culture. The very small chemical shift differences between WT and mutant SOD1 indicate high structural similarity (see Supplementary Fig. 4 ). Full size image The absence or low amounts of E,Zn-SOD1 observed in some fALS-linked mutants suggests a possible detrimental effect of these mutations on some maturation steps of SOD1. To more thoroughly investigate metal uptake, SOD1 fALS mutants that were unable to bind zinc were also analysed in vitro . The protein in the earliest state of folding, that is, apo-reduced (apo-SOD1 SH ) of AV4, G37R, G85R, G93A and I113T, showed signals of the unstructured form also in in vitro NMR spectra ( Supplementary Fig. 5 ) with markedly similar peak patterns as those observed for the same mutants in-cell, suggesting that they are in fact the same species. In addition, a set of more dispersed peaks arising from the native, partially structured apo-SOD1 SH form were also present, with I113T appearing to have the highest ratio of the native form, while the other mutants had little or no native form present ( Supplementary Fig. 5 ). Subsequent titration of the mutants with Zn 2+ revealed that only the native structured form of apo-SOD1 SH can effectively bind the metal. For I113T, A4V, G37R and G93A mutants, the chemical shifts associated with the native, structured form of the apo state were perturbed upon addition of zinc, while the chemical shifts associated with the unstructured form remained unchanged ( Supplementary Figs 5 and 6 ), confirming that the unstructured species is unable to bind zinc. Inductively coupled plasma-atomic emission spectroscopy (ICP-AES) analysis of in vitro samples of apo-G93A mutant incubated with excess of zinc revealed very low metal content (0.11±0.08 equivalent of Zn 2+ per monomer). Thiol alkylation reaction with 4-acetamido-4′-maleimidylstilbene-2,2′-disulfonic acid (AMS) on a fresh cell extract containing apo-G93A mostly in the unstructured state, showed that only the fully reduced species was present ( Fig. 4a ). In addition, the Cβ chemical shift of three out of four cysteines could be measured by NMR directly on a cell extract containing [ 13 C, 15 N]Cys-labelled G93A. The Cβ chemical shifts confirm that all the detected cysteines are reduced ( Fig. 4b ). 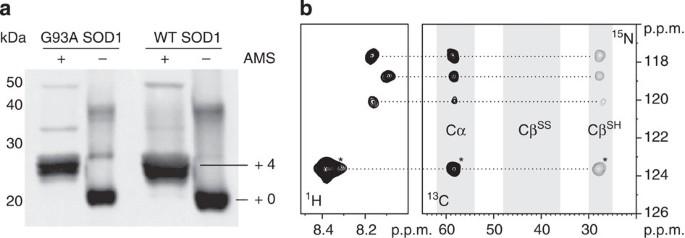Figure 4: The unstructured form of apo-G93A is fully reduced in the cell. (a) Thiol alkylation reaction with AMS on cell extracts containing [13C,15N]Cys-labelled G93A and WT SOD1 expressed in excess of zinc was run on a non-reducing SDS–PAGE and detected with western blot analysis. The band shift corresponds to four linked AMS, indicating that all four cysteines were reduced. (b) 2D projections of a three-dimensional CBCANH NMR experiment, showing that the Cβ chemical shift of three out of four cysteines could be measured, and corresponds to that of reduced cysteines (CβSH), while no signal is detected in the region of the Cβ of oxidized cysteines (CβSS). Cα, CβSSand CβSHregions are showed as light grey areas. The crosspeaks arising from [13C,15N]Cys-labelled glutathione are marked with an asterisk. Figure 4: The unstructured form of apo-G93A is fully reduced in the cell. ( a ) Thiol alkylation reaction with AMS on cell extracts containing [ 13 C, 15 N]Cys-labelled G93A and WT SOD1 expressed in excess of zinc was run on a non-reducing SDS–PAGE and detected with western blot analysis. The band shift corresponds to four linked AMS, indicating that all four cysteines were reduced. ( b ) 2D projections of a three-dimensional CBCANH NMR experiment, showing that the Cβ chemical shift of three out of four cysteines could be measured, and corresponds to that of reduced cysteines (Cβ SH ), while no signal is detected in the region of the Cβ of oxidized cysteines (Cβ SS ). Cα, Cβ SS and Cβ SH regions are showed as light grey areas. The crosspeaks arising from [ 13 C, 15 N]Cys-labelled glutathione are marked with an asterisk. Full size image Unstructured SOD1 observed by NMR is not a soluble oligomer We conducted analytical and semi-preparative gel filtration experiments on in vitro samples of the G93A mutant ( Supplementary Fig. 7a ). Oxidized and reduced samples of apo-G93A were run on an analytical G4000SW XL column to screen for any potentially high molecular weight species, such as the previously characterized soluble oligomeric (SO) species comprised of apo-SOD1 (refs 28 , 34 ). High molecular weight species were not observed in either the oxidized or reduced apo-G93A samples; however, incubation of apo-G93A SH for 96 h at 37 °C resulted in the formation of such a species, albeit at low quantity. The new species eluted at the same volume as the previously characterized SO species when using the same column and incubation times and conditions [34] . Given that the SO species only appeared in small quantities after 96 h of incubation, it is most likely that the unstructured species observed by NMR and the SO species are not the same. Oxidized and reduced samples of apo-G93A were also run on a semi-preparative Superdex HR 10/30 column and peak fractions were collected. NMR analysis of the singular peak observed in the chromatogram for apo-G93A SS revealed that the protein was mostly structured apo-SOD1 SS , while the main peak from the apo-G93A SH chromatogram contained the unstructured form ( Supplementary Fig. 8 ), with both forms having nearly identical elution volumes. To further show the equivalence of the intracellular unstructured species with those observed in vitro , a cleared extract from cells expressing the G93A mutant in excess of zinc was run on the analytical G4000SW XL column using the same experimental conditions ( Supplementary Fig. 7b ). SOD1 was detected by western blot analysis on the collected fractions, and the reconstructed elution profile showed only one peak eluting at the same apparent molecular weight of the in vitro apo-G93A SH sample. Unstructured SOD1 has no secondary structure propensity We subsequently expanded the in vitro characterization of the unstructured species of apo-G93A SH , which was considered representative of the unstructured species of the other mutants owing to the high similarity of both the in-cell and the in vitro 2D NMR spectra ( Fig. 2 and Supplementary Fig. 5 ). By analysing in vitro a U- 13 C, 15 N labelled sample of G93A, we performed a partial backbone sequential assignment. Most of the assigned residues could be remapped on the in-cell NMR spectra of unstructured apo-G93A SH , confirming that the intracellular and the in vitro species are indeed very similar ( Fig. 5 ). Deviations of the chemical shifts from their random coil values indicate the relative tendency of a polypeptide chain to adopt either helical or extended conformations, reflecting therefore the conformational preferences of polypeptide chains with atomic resolution. The secondary structure propensity of unstructured apo-G93A SH was compared with that one of apo WT SOD1 SH and of Cu(I),Zn-SOD1 SS in vitro ( Fig. 6 ). It results that residues located in β-strands in the Cu(I),Zn-SOD1 SS do not have any β structure propensity in unstructured apo-G93A SH , while a high β-strand propensity is still present for the same residues of folded apo WT SOD1 SH . Interestingly, in both unstructured apo-G93A SH and folded apo WT SOD1 SH , the α-helix (residues 130–136) is only transiently populated. 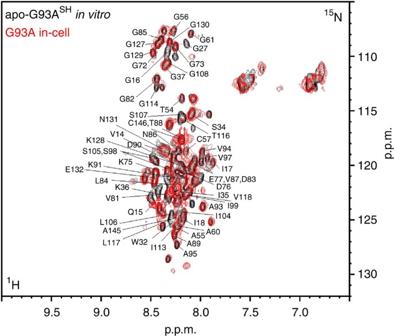Figure 5:In vitroand in-cell NMR spectra of apo-G93ASHshow high chemical shift similarity. Overlay of1H–15N SOFAST HMQC spectra of anin vitrosample of apo-G93ASHSOD1 (black) with an in-cell sample of G93A (red), both acquired at 305 K. For the assigned crosspeaks, the corresponding residue is indicated. Figure 5: In vitro and in-cell NMR spectra of apo-G93A SH show high chemical shift similarity. Overlay of 1 H– 15 N SOFAST HMQC spectra of an in vitro sample of apo-G93A SH SOD1 (black) with an in-cell sample of G93A (red), both acquired at 305 K. For the assigned crosspeaks, the corresponding residue is indicated. 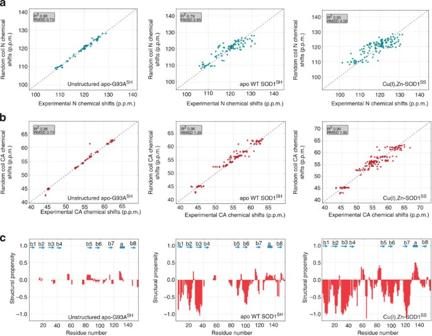Figure 6: The unstructured form of apo-G93ASHdoes not have any β-strand structural propensity. Correlation plots between experimental and predicted N (a) and Cα (b) chemical shifts using random coil libraries56are reported for the unstructured apo-G93ASH, the native, folded apo WT SOD1SHand the fully mature, oxidized Cu(I),Zn-SOD1SS. The fit parameters for the functionf(x)=ax+b using least-square method (R2and root mean square difference (RMSD)) are indicated for each plot;c) the overall secondary structure propensity (SSP) score per residue obtained by using a weighted combination of backbone secondary chemical shifts57is reported for unstructured apo-G93ASH, apo WT SOD1SHand Cu(I),Zn-SOD1SS. Positive SSP values indicate α-helical propensity while negative values correspond to β-strand propensity. Full size image Figure 6: The unstructured form of apo-G93A SH does not have any β-strand structural propensity. Correlation plots between experimental and predicted N ( a ) and Cα ( b ) chemical shifts using random coil libraries [56] are reported for the unstructured apo-G93A SH , the native, folded apo WT SOD1 SH and the fully mature, oxidized Cu(I),Zn-SOD1 SS . The fit parameters for the function f ( x )=a x +b using least-square method ( R 2 and root mean square difference (RMSD)) are indicated for each plot; c ) the overall secondary structure propensity (SSP) score per residue obtained by using a weighted combination of backbone secondary chemical shifts [57] is reported for unstructured apo-G93A SH , apo WT SOD1 SH and Cu(I),Zn-SOD1 SS . Positive SSP values indicate α-helical propensity while negative values correspond to β-strand propensity. Full size image hCCS rescues the impaired zinc-binding step of SOD1 mutants The effect of hCCS in the maturation of SOD1 mutants in living cells was assessed by inducing simultaneous expression of each SOD1 mutant with hCCS in either U- 15 N-labelled or [ 15 N]Cys-labelled medium supplemented with zinc and copper, and by analysing the protein metallation and cysteine redox states. With the exception of the G85R mutant, the fully mature form (Cu(I),Zn-SOD1 SS ) was obtained for each mutant ( Figs 7 and 8 ), while no apo forms, either native or unstructured, were detected ( Supplementary Fig. 9 ), indicating that the SOD1 mutants can reach the mature state when both hCCS and copper are available in the cytoplasm in sufficient amount. A fraction of E,Zn-SOD1 SS was also present for some mutants (namely V7E, G37R, T54R, G93A, I113T, V148I), as well as for WT SOD1 ( Fig. 7 ). Fully mature SOD1 was not observed when mutants were coexpressed with hCCS in the presence of zinc but no copper was supplemented ( Supplementary Fig. 10 ). In these conditions, a mixture of species was generated, mostly E,Zn-SOD1 SH and E,Zn-SOD1 SS , indicating that copper-free hCCS partially restored the zinc-binding step of SOD1 mutants. Together, these results demonstrate that copper is required, together with the coexpression of hCCS, to promote mutant SOD1 maturation, and suggest that hCCS, even without copper, prevents the formation of the unstructured species. 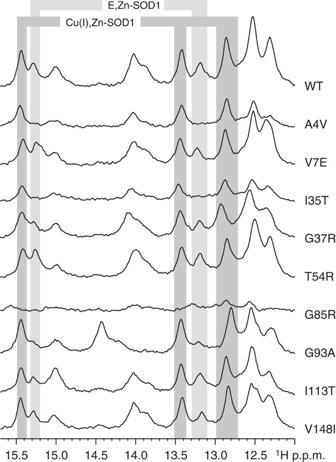Figure 7: In the presence of Cu(I)-hCCS, all SOD1 mutants reach the folded mature state. Histidine regions of1H NMR spectra acquired on human cells coexpressing unlabelled fALS-linked SOD1 mutants together with hCCS, in excess of both zinc and copper. The presence of Cu(I)-hCCS in the cytoplasm allows the formation of mature SOD1 (Cu(I),Zn-SOD1SS) for all mutants, with the exception of G85R. A small amount of E,Zn-SOD1 is still present for some mutants. Histidine protons unambiguously assigned to E,Zn-SOD1 and Cu(I),Zn-SOD1 species are indicated in light grey and dark grey, respectively. Figure 7: In the presence of Cu(I)-hCCS, all SOD1 mutants reach the folded mature state. Histidine regions of 1 H NMR spectra acquired on human cells coexpressing unlabelled fALS-linked SOD1 mutants together with hCCS, in excess of both zinc and copper. The presence of Cu(I)-hCCS in the cytoplasm allows the formation of mature SOD1 (Cu(I),Zn-SOD1 SS ) for all mutants, with the exception of G85R. A small amount of E,Zn-SOD1 is still present for some mutants. Histidine protons unambiguously assigned to E,Zn-SOD1 and Cu(I),Zn-SOD1 species are indicated in light grey and dark grey, respectively. 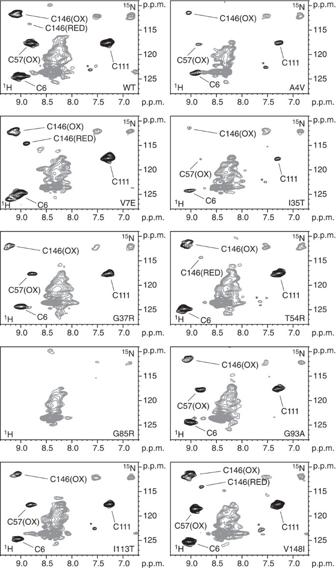Figure 8: Cu(I)-hCCS catalyses disulfide bond formation on SOD1 mutants. 1H–15N SOFAST-HMQC spectra of cells expressing [15N]Cys-labelled fALS SOD1 mutants together with hCCS, in the presence of both zinc and copper, showing that Cu(I)-hCCS catalyses the formation of the SOD1 intramolecular disulfide bond. SOD1 cysteine crosspeaks (black) are labelled. For Cys57 and Cys146 crosspeaks, the oxidation state is also indicated. A crosspeak from [15N]Cys-labelled hCCS is marked with an asterisk. Signals arising from cellular background are shown in grey. The cysteine assignments of fALS SOD1 mutants are taken from that of WT SOD1 cysteines, which were obtained by comparingin vitrospectra of reduced and oxidized [15N]Cys-labelled SOD1 with the available backbone assignments4,58. Full size image Figure 8: Cu(I)-hCCS catalyses disulfide bond formation on SOD1 mutants. 1 H– 15 N SOFAST-HMQC spectra of cells expressing [ 15 N]Cys-labelled fALS SOD1 mutants together with hCCS, in the presence of both zinc and copper, showing that Cu(I)-hCCS catalyses the formation of the SOD1 intramolecular disulfide bond. SOD1 cysteine crosspeaks (black) are labelled. For Cys57 and Cys146 crosspeaks, the oxidation state is also indicated. A crosspeak from [ 15 N]Cys-labelled hCCS is marked with an asterisk. Signals arising from cellular background are shown in grey. The cysteine assignments of fALS SOD1 mutants are taken from that of WT SOD1 cysteines, which were obtained by comparing in vitro spectra of reduced and oxidized [ 15 N]Cys-labelled SOD1 with the available backbone assignments [4] , [58] . Full size image In the in-cell NMR experiments, SOD1 and hCCS were coexpressed in the presence of copper and oxygen, therefore the two steps of CCS-dependent maturation—copper transfer and disulfide bond oxidation—could not be separated. To examine these steps separately, and determine if fALS mutations affect the kinetics of either process, we characterized the interaction of Cu(I)-hCCS with the E,Zn-hSOD1 SH form of WT and mutants by in vitro NMR experiments. Anaerobic incubation of E,Zn-hSOD SH WT and fALS mutants V7E, G37R, T54R, G85R, G93A, I113T and V148I with Cu(I)-hCCS resulted in the formation of the Cu,Zn-hSOD1 SH , with 100% copper incorporation for all the fALS mutants, and an apparent rate similar to that of the WT protein ( Supplementary Fig. 11a ). Once fully copper loaded, exposure to air produced the fully mature Cu,Zn-hSOD1 SS form, with rates comparable to that of WT SOD1 still in the presence of hCCS ( Supplementary Fig. 11b ). Only the T54R mutant protein resulted in a considerably slower oxidation of the C57-C146 disulfide bond (see Supplementary Fig. 12 for a detailed analysis), although its oxidation was faster in the presence of Cu(I)-hCCS than without. For mutants where the unstructured apo species was present together with E,Zn-hSOD1 SH (G37R, G85R and G93A) the unstructured apo species was unaffected by in vitro addition of Cu(I)-hCCS (for example G85R, Supplementary Fig. 13 ). The maturation process of a set of fALS-linked SOD1 mutants was analysed in their physiological environment, by comparing the distribution of species produced by the cells in different metal abundance, with respect to that of WT SOD1 in the same conditions, and the role of hCCS in promoting mutant SOD1 maturation was investigated. Many of the fALS mutants analysed here appeared to form an unstructured species when overexpressed in cells with only endogenous levels of hCCS ( Fig. 9 ). This unstructured SOD1 species was observed both in-cell and in vitro , and is unaffected by the presence of excess zinc: supplementation of zinc in the media of cells expressing fALS mutants with only endogenous hCCS did not affect the signals associated with the unstructured species, nor, in the case of the in vitro experiments, did direct addition of zinc to fALS mutant samples, indicating that, in this form, SOD1 is unable to bind zinc. 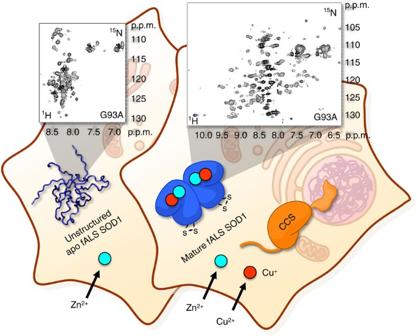Figure 9: Illustration showing the different intracellular states observed for some SOD1 fALS mutants. Left, a subset of SOD1 fALS mutants accumulates in the cells in an unstructured form (blue), which is unable to bind zinc (cyan) even when the latter is supplemented in excess. Right, coexpression of the copper chaperone hCCS (orange) and incubation with excess copper (dark orange) restore the correct maturation pathway, and Cu(I),Zn-SOD1SSis formed. In-cell NMR spectra of G93A SOD1 in the two states are shown as an example. Figure 9: Illustration showing the different intracellular states observed for some SOD1 fALS mutants. Left, a subset of SOD1 fALS mutants accumulates in the cells in an unstructured form (blue), which is unable to bind zinc (cyan) even when the latter is supplemented in excess. Right, coexpression of the copper chaperone hCCS (orange) and incubation with excess copper (dark orange) restore the correct maturation pathway, and Cu(I),Zn-SOD1 SS is formed. In-cell NMR spectra of G93A SOD1 in the two states are shown as an example. Full size image The unstructured species was not observed for the same mutants, with the exception of G85R, when hCCS was coexpressed in the presence of copper and zinc. In this case, only mature SOD1 forms were detected ( Fig. 9 ). This demonstrates that the unstructured species does not form when the hCCS-dependent SOD1 maturation mechanism is intact and can readily convert the immature protein to the metallated dimeric protein. Coexpression of hCCS in the absence of copper also prevented, at least in part, the formation of the unstructured species, and promoted the formation of a mixture of E,Zn-SOD1 SH and E,Zn-SOD1 SS . These observations point to a possible molecular chaperone function of hCCS, as already proposed [45] , [46] , which would transiently interact with apo-SOD1 SH and stabilize it long enough to allow zinc binding to occur. In the case of G85R no mature protein was formed, even in the presence of Cu(I)-hCCS. Likely, the reduced affinity of G85R for zinc caused the intracellular accumulation of unstructured form even in the presence of hCCS and, thus, the formation of the metallated dimeric protein did not occur. According to the proposed folding model of SOD1, the native, partially folded, apo monomer is in equilibrium with an unfolded monomeric state [47] , [48] . For some of the fALS mutant proteins, this equilibrium has been shown to be shifted towards the unfolded monomeric form [49] , [50] , which has also been suggested to be the starting material for the potentially toxic oligomeric species [42] , [49] . This unfolded monomer is likely identical to the SOD1 polypeptide that exits the ribosome, and should shift to the folded, dimeric E,Zn-SOD1 SH form upon zinc binding [50] . Although the unfolded monomeric state has also been reported to have a significantly reduced binding affinity for zinc [51] , this form cannot be the same as the unstructured species identified here, as the latter is unable to bind zinc and does not convert to the folded monomeric conformation, which would bind zinc with high affinity. Therefore, on the basis of these observations, we propose that the unstructured species observed here is generated from the monomeric apo species, which evolves towards a non-correct, irreversible arrangement. Indeed, the addition of zinc and interaction with hCCS do not induce its folding back to the native form in vitro . Formation of the unstructured species is relatively slow, as the presence of hCCS is able to prevent its accumulation in the cell. Thus, the current study supports a model whereby, due to a higher propensity to remain unfolded, fALS mutations result in an increased population of the unfolded monomeric apo form, which is the starting material for the irreversible formation of the unstructured species. This species could then give rise, at a later stage, to the potentially toxic oligomeric species, and eventually to the aggregation products that are the hallmark of the SOD1-linked ALS disease. The unstructured species, observed here by in-cell and in vitro NMR for the first time, may have been previously reported in other works, in which irreversibly unfolded species, originating from a common apo-SOD1 disulfide reduced form, have been proposed [50] , [52] . An intracellular structural approach, such as in-cell NMR, is therefore necessary to understand the intricate protein misfolding pathways that underlie many degenerative diseases. In this study, we have characterized the critical maturation steps of a number of fALS-linked SOD1 mutants directly in living human cells by in-cell NMR, coupled with in vitro characterization. For a subset of fALS mutants, we have observed the presence of an unstructured species, unable to bind zinc or interact with hCCS, which is likely a precursor to potentially toxic aggregation products that have been linked with the disease. By in-cell NMR, we have also shown that the coexpression of hCCS prevents the formation of the unstructured species in the cell, and that Cu(I)-hCCS is able to restore the correct maturation of mutant SOD1. These results suggest that the detrimental effects of the fALS mutations can be mitigated by hCCS. We have shown that hCCS, by interacting with the immature fALS SOD1 mutants, could exert a role of molecular chaperone for SOD1, as already suggested [45] , [46] , independent of its role as a copper chaperone, thus modulating the formation of toxic species precursor. Gene cloning for in-cell NMR SOD1 fALS mutants (with the exception of G85R) were obtained by site-directed mutagenesis on the WT gene inside the pTH34 vector. The mutated genes were subcloned in the pHLsec vector between EcoRI and XhoI restriction enzymes [53] . All the clones were verified by DNA sequencing. Cell culture and transfection HEK293T (ATCC CRL-11268) cells were maintained in Dulbecco’s Modified Eagle’s medium (DMEM; high glucose, D6546, Sigma) supplemented with L -glutamine, antibiotics (penicillin and streptomycin) and 10% FBS (Gibco) in uncoated 75-cm 2 plastic flasks and incubated at 310 K, 5% CO 2 in a humidified atmosphere. Cells were transiently transfected with the pHLsec plasmid containing the cDNA using polyethylenimine (PEI). For expression of WT and mutant SOD1 alone, the DNA was incubated with PEI in 5 ml serum-free DMEM for 20 min, in a 1:2 weight ratio (25 μg per flask DNA, 50 μg per flask PEI). For coexpression of mutants SOD1 and hCCS, cells were transfected with plasmids containing both constructs in a 1:1:2 (SOD1:CCS:PEI) weight ratio. Commercial DMEM medium was used for unlabelled in-cell NMR samples; BioExpress6000 medium (CIL) was used for U- 15 N-labelling; for selective [ 15 N]cysteine labelling, a reconstituted medium was prepared following the DMEM (Sigma)-reported composition, in which [ 15 N]cysteine was added together with all the other unlabelled components. Expression media were supplemented with 2% FBS and antibiotics. Zn(II) was supplemented as ZnSO 4 , which was added to the expression media to a final concentration of 10 μM immediately after transfection. Cu(II) was supplemented as CuCl 2 , added to expression media to a final concentration of 50 μM after 48 h of protein expression, and the cells were further incubated for 24 h. Protein expression levels were monitored by western blot analysis. SOD1 mutants were stained with a rabbit polyclonal anti-SOD1 antibody (BioVision: catalogue #: 3458-100, diluted to 1 μg ml −1 ). Goat anti-rabbit IgG (whole molecule)-peroxidase secondary antibody (Sigma:A0545) was used, diluted at 1:80,000. For detection, LiteAblot EXTEND chemiluminescent substrate (EuroClone) was used. In-cell NMR experiments Cell samples for in-cell NMR were prepared following a reported protocol [10] . Briefly, transfected HEK293T cells were detached with trypsin, suspended in DMEM+10% FBS, washed once with phosphate-buffered saline and re-suspended in one pellet volume of DMEM supplemented with 90 mM glucose, 70 mM HEPES for increased pH stability and 20% D 2 O. The cell suspension was transferred in a 3 mm Shigemi NMR tube and cells were allowed to settle on the bottom. 1D 1 H and 2D 1 H– 15 N SOFAST HMQC NMR experiments were acquired using a 950-MHz Bruker Avance III spectrometer equipped with a CP TCI CryoProbe at 305 K. The total acquisition time for each cell sample ranged from 1 to 2 h. The supernatant of each cell sample was checked in the same experimental conditions to exclude protein leakage. Cell viability before and after NMR experiments was assessed by trypan blue staining. After the experiments, cells were suspended in phosphate-buffered saline-EDTA buffer and lysed by freeze–thaw method. Upon centrifugation, the supernatant containing the cell extract was collected for further analysis. In vitro experiments Wild-type and SOD1 fALS mutants were expressed in the Escherichia coli ( E. coli ) Origami pLys (Novagen) cells. The proteins were synthesized after an induction with 0.7 mM isopropyl β- D -thiogalactopyranoside (IPTG) for 16 h. Cells were ruptured by sonication and the proteins purified to homogeneity using a HiTrap chelating HP column (Amersham Pharmacia Biosciences) charged with Ni(II). The GB1/His tag was cleaved with AcTEV. The digested protein was concentrated by ultrafiltration and loaded in a 16/60 Superdex 75 chromatographic column (Amersham Pharmacia Biosciences). The fractions showing a single component by SDS–polyacrylamide gel electrophoresis (SDS–PAGE) were collected, and the protein concentration was measured using the Bradford protein assay. The hCCS gene was amplified by PCR, cloned into the Gateway pDONR 221 Entry vector (Invitrogen), and subcloned into the pTH27 Destination vector by a Gateway cloning system (Invitrogen) to generate an amino (N)-terminal, His fused protein. The protein was expressed in E. coli BL21(DE3) Codon Plus RIPL cells (Stratagene). Protein expression was induced with 0.7 mM IPTG for 16 h. ZnSO 4 was added in the culture to a final concentration of 1 mM. Purification of hCCS protein was performed using a HiTrap chelating HP column charged with Ni(II). The His tag was cleaved with AcTEV. The digested protein was concentrated by ultrafiltration and loaded in a 16/60 Superdex 75 chromatographic column to separate hCCS from the N-terminal His tag. The fractions showing a single component by SDS/PAGE were collected, and the protein concentration was measured using the Bradford protein assay. For 15 N labelled proteins, the cells were grown in M9 minimal media supplemented with ( 15 NH 4 ) 2 SO 4 . For titration of apo-reduced fALS mutants (AV4, G37R, G85R, G93A and I113T) with zinc, 15 N-labelled apo-proteins were prepared by dialyzing the proteins against 10 mM EDTA in 50 mM sodium acetate (pH 3.8). EDTA was removed by extensive dialysis against 100 mM NaCl in the same buffer and then against acetate buffer alone, gradually increasing the pH from 3.8 to 5.5. The apo-proteins were then reduced with 200 mM dithiothreitol (DTT) and washed with 100 mM sodium phosphate buffer, 100 mM NaCl at pH 6.0. The samples (80–120 μM) were then titrated with a stock solution of 10 mM ZnCl 2 and monitored by 1 H– 15 N SOFAST HMQC until the formation of the E,Zn-hSOD1 species was observed. The backbone assignments of E,Zn-hSOD1 and Cu,Zn-hSOD1 have been previously published [54] , [55] . For incubation of E,Zn-reduced WT and fALS mutants, with the exception of the A4V and I35T, with unlabelled Cu(I)-hCCS, E,Zn-oxidized samples obtained after expression and purification were reduced using DTT and washed with 100 mM sodium phosphate buffer, 100 mM NaCl at pH 6.0. Excess Cu(I)-hCCS was then added to SOD1 proteins (80–120 μM) and monitored for copper transfer using a series of 1 H– 15 N SOFAST HMQC experiments. Oxidation rates were then monitored in the same fashion after exposure of the sample to air for 10 min. E,Zn-reduced WT and T54R were also titrated with the acetonitrile complex of copper(I), [Cu I (CH 3 CN) 4 ] and exposed to air to monitor the rate of oxidation of the Cu,Zn-hSOD1 SH species in the absence of hCCS. A4V and I35T were not examined in this fashion, as the intensity of the NMR signals associated with the folded regions was below the detection limit. All sample preparations were carried out in a N 2 atmosphere chamber, and the NMR tubes were sealed before removing them from the chamber. All NMR samples contained 10% v/v D2O for NMR spectrometer lock. In vitro NMR experiments were recorded at 298 K at Bruker Avance 800 and 900 MHz spectrometers, equipped with cryo-cooled probes. Size exclusion chromatography Twenty microlitres of apo-G93A SS , apo-G93A SH and apo-G93A SH incubated at 37 °C for 96 h (80–120 μM) were analysed by gel filtration on a G4000SW XL (Tosoh Bioscience) column. One hundred microlitres of apo-G93A SS and apo-G93A SH (80–120 μM) were also analysed on a Superdex 75 HR 10/30 (Amersham Pharmacia Biosciences) column. Both columns were preequilibrated at room temperature with 100 mM sodium phosphate buffer, 100 mM NaCl at pH 6.0. Flow rates of 0.8 and 0.5 ml min −1 were used, respectively. Twenty microlitres of extract from cells expressing G93A was also examined by gel filtration on a G4000SW XL column, using the same experimental conditions. Three hundred microlitre fractions were collected and analysed by western blot analysis. Zinc content determination Samples of the unstructured form of apo-G93A SH collected from the Superdex 75 HR 10/30 column were treated with excess zinc and thoroughly washed with buffer. The zinc content of each sample was measured by ICP-AES on a ICP-AES VARIAN 720-ES spectrometer. The protein concentration was calculated from the UV absorbance measured with a NanoVue (GE Healthcare), using the SOD1 monomer molar extinction coefficient (7,400 l mol −1 cm −1 at 265 nm). Reaction with AMS Reaction with AMS was performed directly on cell lysate samples in oxygen-free conditions. One hundred and eighty microlitres of cell lysate was precipitated with 10% trichloroacetic acid, washed with 150 μl acetone and re-suspended in 100 μl 100 mM Tris buffer, pH 7+2% SDS. Twenty microlitres of the mixture obtained was incubated for 1 h at 37 °C with 40 mM AMS, and finally run on a non-reducing SDS–PAGE. The gel was electroblotted on to a nitrocellulose membrane and probed with a rabbit anti-SOD1 antibody (Abcam ab16831) and with a goat anti-rabbit IgG (whole molecule)-peroxidase secondary antibody (Sigma:A0545). How to cite this article: Luchinat, E. et al . In-cell NMR reveals potential precursor of toxic species from SOD1 fALS mutants. Nat. Commun. 5:5502 doi: 10.1038/ncomms6502 (2014).